Stress-induced chemical waves in sediment burial diagenesis Lateral metre-scale periodic variations in porosity and composition are found in many dolomite strata. Such variations may embed important information about dolomite formation and transformation. Here we show that these variations could be fossilized chemical waves emerging from stress-mediated mineral-water interaction during sediment burial diagenesis. Under the overlying loading, crystals in higher porosity domains are subjected to a higher effective stress, causing pressure solution. The dissolved species diffuse to and precipitate in neighbouring lower porosity domains, further reducing the porosity. This positive feedback leads to lateral porosity and compositional patterning in dolomite. The pattern geometry depends on fluid flow regimes. In a diffusion-dominated case, the low- and high-porosity domains alternate spatially with no directional preference, while, in the presence of an advective flow, this alternation occurs only along the flow direction, propagating like a chemical wave. Our work provides a new perspective for interpreting diagenetic signatures in sedimentary rocks. Owing to their geological importance, dolomite formations have been intensively characterized, both physically and chemically. Recent high-resolution sampling (with a sampling interval of 0.3 m) has revealed complex nested patterns of lateral porosity and permeability variations in dolomite strata [1] ( Fig. 1 ). Three scales of lateral variability are documented, including a near-random component at <0.3 m, a short-range correlation structure of 4.0–6.7 m and longer periodic structures with wavelengths up to 12.2 m (ref. 2 ). The porosity usually oscillates in a range between 10 and 25%, while the permeability could vary by a factor of ~100 ( Supplementary Fig. S1 ). Trace element contents and isotopic compositions vary in a similar manner [1] ( Supplementary Fig. S1 ). These oscillations appear to be common in many dolomite strata [3] , [4] , [5] , [6] , [7] . 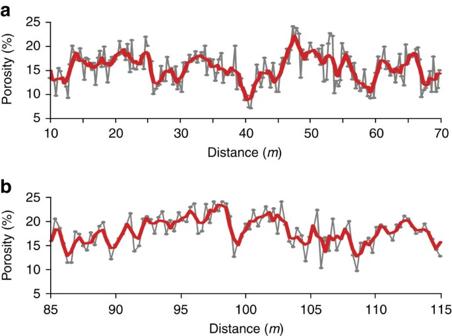Figure 1: Lateral porosity variations in dolomite. Porosity measurements were performed over 60- and 30-m transects, respectively, in Madison dolograinstone (a) and dolowackestone (b). Solid red lines are three-point moving averages. Data are taken from ref.2. Figure 1: Lateral porosity variations in dolomite. Porosity measurements were performed over 60- and 30-m transects, respectively, in Madison dolograinstone ( a ) and dolowackestone ( b ). Solid red lines are three-point moving averages. Data are taken from ref. 2 . Full size image A mechanistic understanding of the origin of such oscillations is of manifold significance. First of all, these oscillations may embed important information about dolomite formation and transformation, and a mechanistic understanding is required to decode the embedded information. It has been suggested that such oscillations might have formed during or after dolomitization [1] , [8] . However, the actual mechanism remains unknown. Furthermore, the existence of these variations raises a serious question about the validity of the existing field sampling schemes that tend to use sparse spot samples as proxies for interpreting ancient geologic environments [1] . A reliable interpretation must account for the lateral heterogeneity in an individual dolomite stratum, based on a clear understanding of the underlying physical and chemical processes. In addition, a mechanistic understanding is also crucial for developing predictive tools for better quantification of spatial heterogeneity in a subsurface reservoir. Such tools are highly desirable for many reservoir engineering applications, as such heterogeneity is known to have a direct impact on pore connectivity, fluid flow patterns and therefore the overall performance of a subsurface reservoir [4] , [6] . In this article, we propose a mechanism that can account for all the main features of lateral physical and chemical variations in dolomite. The proposed mechanism is based on the concept of geochemical self-organization and chemical waves [9] , [10] . Using a linear stability analysis, we show that the observed lateral variations could autonomously emerge from stress-mediated mineral dissolution and precipitation during sediment burial diagenesis. These variations provide rich information about ancient geologic environments for dolomite formation and transformation. The proposed mechanism is expected to be universal for all sediments. Our work provides a new perspective for interpreting petrophysical and chemical signatures in sedimentary rocks. Effective stress–porosity feedback Self-organization requires a positive feedback among physical and chemical processes involved in a system [11] . To illustrate the concept, let us consider a post-dolomitization scenario, in which a layer of dolomite with uniform depositional properties (that is, a uniform facies) and a thickness H undergoes burial diagenesis under a vertical loading σ 0 ( Fig. 2 ). The change in porosity ( φ ) can be described by: where t is time; v m is the molar volume of dolomite [CaMg(CO 3 ) 2 ] (cm 3 mol −1 ); and R d is the mineral dissolution rate (mol cm −3 bulk rock s −1 ). The first term on the right side represents the porosity reduction due to mechanical compaction. The second term denotes the porosity increase due to mineral dissolution. The dissolution rate R d is assumed to follow the first-order kinetics: where k is the reaction rate constant (cm 3 solution cm −2 s −1 ); S is the specific reactive surface area (cm 2 cm −3 solid); C is the concentration of dissolved dolomite species (mol cm −3 solution) (for simplicity, they are here represented by a single equivalent species); and C s is the solubility of dolomite, assumed to be a function of the effective stress σ (bar) to which mineral grains are subjected [12] ; Δ v is the molar volume change of dolomite dissolution reaction (cm 3 mol −1 ); R is the gas constant (cm 3 bar mol −1 K −1 ); T is the temperature (K); and C e 0 is the solubility of dolomite under no stress. The term (1− φ ) is the volumetric fraction of solid in the bulk rock (cm 3 solid cm −3 bulk rock). 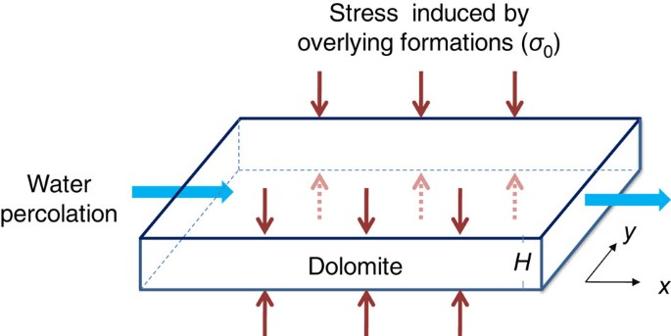Figure 2: Schematic representation of the modelled system. A dolomite stratum of thicknessHis subject to a vertical stress (σ0) caused by overlying geologic formations. Under certain conditions, stress-induced mineral dissolution and precipitation causes lateral porosity differentiation. Water percolation may affect the porosity pattern formed. Figure 2: Schematic representation of the modelled system. A dolomite stratum of thickness H is subject to a vertical stress ( σ 0 ) caused by overlying geologic formations. Under certain conditions, stress-induced mineral dissolution and precipitation causes lateral porosity differentiation. Water percolation may affect the porosity pattern formed. Full size image Lateral porosity differentiation occurs when the chemical reaction term, v m R d , overtakes the compaction rate, ((1− φ )/ H ) dH / dt , in equation (1) ( Fig. 3 ). In this case, a positive feedback between mineral dissolution and stress becomes possible: crystal grains in a higher porosity domain within the layer are subjected to a higher effective stress than those in a lower porosity domain, thus resulting in pressure solution. The dissolved species diffuse to and precipitate in neighbouring lower porosity domains, further reducing the porosity in these domains. As shown below, this positive feedback leads to a lateral porosity differentiation within the dolomite layer. The differentiation would tend to occur in a consolidated sediment stratum comprising rigid mineral grains, in which mechanical compaction would be relatively small. For a rigid grain, such as a dolomite crystal, the influence of the exerting stress would extend to the whole grain, and dissolution thus occurs across the whole grain surface, especially on the pore surface, where the dissolved species can be easily transported away. 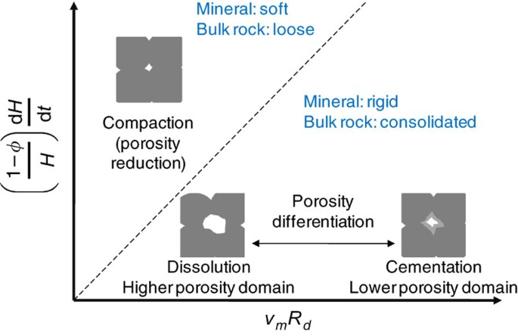Figure 3: Conditions for stress-induced porosity differentiation in a buried sediment stratum. Porosity differentiation occurs when the chemical reaction rate,vmRd, overtakes the mechanical compaction rate, ((1−φ)/H)dH/dt. This differentiation preferentially occurs in a consolidated sediment stratum comprising rigid mineral phases. Figure 3: Conditions for stress-induced porosity differentiation in a buried sediment stratum. Porosity differentiation occurs when the chemical reaction rate, v m R d , overtakes the mechanical compaction rate, ((1− φ )/ H )d H /d t . This differentiation preferentially occurs in a consolidated sediment stratum comprising rigid mineral phases. Full size image Stress-mediated reactive transport For simplicity, we assume that the mechanical compaction term is negligible as compared with the chemical reaction term. The porosity evolution of the dolomite layer is depending on three unknowns ( C, P and φ ) and governed by where P is the hydraulic head (cm). The effective diffusion coefficient D ( φ ) (cm 2 s −1 ) and the hydraulic conductivity K ( φ ) (cm s −1 ) are described by respectively [13] , [14] , [15] , where D 0 is the diffusion coefficient of dissolved species in solution, and both m (≈2) (ref. 14 ) and K 0 are constants. The effective stress to which mineral grains are subjected at a spatial point ( X , Y ) is expected to depend on the overlying loading σ 0 , the local porosity and the porosity distribution in the neighbourhood (that is, the rock texture in the neighbourhood). We define a texture descriptor ψ ( X,Y,t ) as a weighted average of porosity in the neighbourhood: where K r is a kernel function with The kernel function is isotropic and independent of location, and vanishes as X − X ′→∞ or Y − Y ′→∞. Based on this symmetry argument, by expanding the term φ in equation (6) into a Taylor's series and collecting the linear and second-order terms, we obtain (see Methods ): where B is a constant. We then assume that the effective stress σ is proportional to the overlying loading σ 0 and some function of ψ , f ( ψ ). where α is a proportionality constant. To ensure that mineral grains in a higher porosity domain is subjected to a higher effective stress, it is required that One reasonable choice for function could be: f ( ψ )=1/1− ψ . The effective stress would then be inversely proportional to the ratio of cross-sectional area of solid to bulk rock. Given a typical porosity value in dolomite (~15%) ( Fig. 1 ), the function chosen can be further simplified: f ( ψ )=1/(1− ψ )≈1+ ψ . Scaling and asymptotic analysis Equations (2–8) form a closed system that describes lateral porosity evolution in a single dolomite layer during burial diagenesis. To delineate the relative importance of each term in the equations, we scale the equations by choosing appropriate time and length scales, a typical dissolved species concentration and a typical hydraulic head so that each variable in the equations has a magnitude of one. From equations (2), (7) and (8), we choose the typical dissolved species concentration ( [Cmacr ] ) to be the solubility of dolomite under a uniformly distributed initial porosity ( φ o ) and a given overlying loading ( σ o ): where . As porosity evolution due to mineral dissolution and precipitation is of our main interest, the relevant time scale would be the one over which a significant change in porosity could occur. The time scale ( T ) is thus chosen to be: obtained by scaling equations (2) and (5). Similarly, the length scale ( L ) and the typical hydraulic head ( [Pmacr] ) and to make both the diffusion term and the advective term in equation (3) comparable with the chemical reaction term so that they can interplay with each other. Accordingly, the other variables and the related mathematical operators can be scaled as follows: y = Y / L , Equations (2–8) can then be cast into a set of dimensionless scaled equations: where These equations show that the system under consideration has dual time scales: T (the long time scale) and ɛT (the short time scale), which is a common feature of many rock–water interaction systems. To study the porosity evolution, we have to use the long time scale T . Given the typical value of v m (=64 cm 3 mol −1 , ref. 16 ) and [Cmacr ] (≈10 −6 mol cm −3 , ref. 17 ), the parameter ɛ is typically very small (<10 −4 ). Therefore, the left-hand side terms in equations (10) and (11) are negligible. These three equations thus can provide solutions to porosity evolution on long time scales, given the three unknowns ( C, P and φ ) of the general case. Linear stability analysis We now perform a linear stability analysis of equations (9–11) to determine the geometry and wavelength of lateral porosity oscillations (details in Methods). We first solve the equations for their steady-state solution: φ s = φ 0 , c s =1 and where v is a scaled fluid flow velocity. We then linearize the equations and introduce a small perturbation around the steady-state solution. Finally, we obtain the following dispersion equations describing the growth rate ( ζ ) of a perturbation of a wave number vector ( ω 1 , ω 2 ): where η = f ′( φ s ). The real part of ζ , Re ( ζ ), represents the actual growth rate of a perturbation, while the imaginary part Im ( ζ ) indicates a temporal oscillation of a spatial pattern. A positive Re ( ζ ) value means that the perturbation with the corresponding wave number tends to grow with time, leading to the emergence of a spatially repetitive pattern [18] . The wave number vector ( ω max ,1 ω max ,2 ) corresponding to the maximum Re ( ζ ) dictates the periodicity (or the spacing) of a pattern actually formed. As indicated in equation (12), the preferred wave number vector ( ω max ,1 ω max ,2 ) is independent of both θ and η . Thus, the choice of the actual form of function f ( ψ ) in equation (8) has no effect on the periodicity of the pattern formed as long as that is, as long as the positive feedback between the effective stress and the porosity is maintained. The linear stability analysis demonstrates that periodic lateral oscillations in porosity can autonomously emerge from the stress-induced instability of sediment burial diagenesis, as indicated by the existence of positive Re ( ζ ) values for certain waves numbers ( Fig. 4 ). In a no-flow case, Re ( ζ ) is a function only of with no directional preference, implying the formation of a spatially isotropic pattern. As Im ( ζ )=0 with no flow, the chemical wave formed would be stationary. In contrast, in a flow case, ω max ,2 =0, that is, an infinite wavelength in Y -direction, indicating that any periodic oscillations in the Y -direction are suppressed, causing a symmetry breakdown. The repetitive patterns can thus form only along the flow direction. With flow, Im ( ζ ) can be non-zero, implying that the porosity at each spatial point would oscillate with time. In that case, the stripes of low- and high-porosity domains would slowly move downstream along the flow path, forming a propagating chemical wave. A careful evaluation of equation (12) indicates that the transition from an isotropic pattern to a stripe pattern occurs when the scaled flow velocity ( v ) is greater than 0.1, corresponding to an actual velocity of ~2 cm per year with the following estimated parameter values: D 0 =10 −4 cm 2 s −1 , k =10 −10 cm 3 solution cm −2 s −1 , S =10 cm 2 cm −3 solid and φ 0 =0.15 (see below for a detailed discussion on the range of parameter values). Therefore, careful characterization of lateral heterogeneity in a dolomite layer may provide rich information about paleo-hydrologic environments for dolomite formation and transformation. 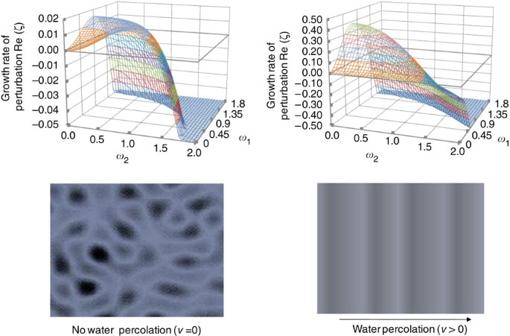Figure 4: Periodic lateral porosity differentiation predicted from a linear stability analysis. The wave number with the maximum growth rate,ωmax, determines the scale of the emerging pattern. As illustrated schematically in the lower panel, in a no-flow case, patterns form with no directional preference (left)whereas in a flow-dominated case patterns tend to form only along the flow path and those in other directions are suppressed (right) (ωmax,1>0,ωmax,2=0), causing the pattern symmetry to break down. Following parameter values are used in the analysis:θ=1,η=1.4,φs=0.15,β=0.5,m=2 andv=0 (left) or 1 (right). The illustration in the lower left panel was modified from ref.6. Figure 4: Periodic lateral porosity differentiation predicted from a linear stability analysis. The wave number with the maximum growth rate, ω max , determines the scale of the emerging pattern. As illustrated schematically in the lower panel, in a no-flow case, patterns form with no directional preference (left) whereas in a flow-dominated case patterns tend to form only along the flow path and those in other directions are suppressed (right) ( ω max, 1 >0, ω max, 2 =0), causing the pattern symmetry to break down. Following parameter values are used in the analysis: θ =1, η =1.4, φ s =0.15, β =0.5, m =2 and v =0 (left) or 1 (right). The illustration in the lower left panel was modified from ref. 6 . Full size image The wavelength of porosity oscillations ( L p =2 πL / ω max ) can be estimated from (see Methods ): for a no-flow case for a flow case with v >0.1 Parameter β characterizes the degree of sediment consolidation (that is, the mechanical strength of bulk sediment). The wavelength increases with sediment mechanical strength, diffusion coefficient and flow velocity, and decreases with mineral dissolution rate. For a no-flow case, taking the typical parameter values for dolomite: β =~1.0, D 0 =~10 −4 −10 −3 cm 2 s −1 (accounting for a possible effect of elevated temperature), k =10 −10 −10 −8 cm 3 solution cm −2 s −1 (using a dolomite dissolution rate of 10 −14 –10 −16 mol cm −2 s −1 (ref. 17 ), and assuming a typical concentration of dissolved species of 10 −6 mol cm −3 (ref. 17 )), S =10−100 cm 2 cm −3 solid and φ 0 =0.15, we estimate the wavelength of the pattern to be 0.3–30 m, consistent with field observations [1] , [2] . Accordingly, the time scale for the predicted porosity differentiation is estimated to be 5×10 2 –5×10 5 years. For a flow case with a typical flow rate of 0.1–20 cm per year [19] , the scaled flow rate ( v ) is estimated to be 0.0001–1. However, as discussed above, the effect of flow on pattern formation becomes significant only when v >0.1. Given that in equation (15), the scale of a pattern formed in a flow case is expected to be on the same order of magnitude as that in a no-flow case, but the geometry of the pattern will be very different. With or without flow, as the sediment undergoes progressive burial diagenesis, newly formed chemical waves may superimpose on the relics of early ones, resulting in complex nested lateral porosity variations. Petrographic observations support our model predictions. Cathodoluminescence images of Mississippian dolomites that exhibit lateral patterns suggest that cement overgrowths on dolomite crystals are common in low-porosity samples while high-porosity samples from the same bed show little dolomite cementation or even dissolution ( Supplementary Fig. S2 ). These features are typically attributed to rock–water interaction processes, but why the abundance of cements would vary laterally on the metre scale is not explained by that traditional interpretation. Our model provides a logical explanation for these lateral variations. Differential mineral dissolution and cementation in different domains are a natural outcome of the proposed self-organization phenomenon. Furthermore, as mentioned above, a stress-induced chemical wave may evolve with time and propagate along a flow path. We would then expect that multiple stages of cementation or dissolution may occur at the same locality in a dolomite layer even under a single-flow regime with a constant fluid composition. This seems consistent with the widespread occurrence of luminescent zonation of dolomite cement. Such zonation has long been interpreted to record varying compositional and/or Eh changes of advecting fluids [20] , [21] . Our model also provides a reasonable explanation for the associated variations in chemical and isotopic signatures [1] ( Supplementary Fig. S1 ). In higher porosity domains, dolomite dissolves, releasing the contained trace elements into pore water. The released trace elements are reincorporated into newly precipitated dolomite cements in lower porosity domains. Consequently, the elements with partitioning coefficients >1 tend to be enriched in these cements, while those with partitioning coefficients <1 are depleted [22] . Bulk-rock geochemical analyses should thus show higher Fe and Mn, and lower Sr, in lower porosity domains. These predictions seem relatively well confirmed by field observations given the dynamic nature of the system that our model reveals. As shown in Supplementary Figure S1 , the contents of trace elements in dolomite oscillate with the similar periods as porosity, with Fe and Mn varying roughly antipathetically and Sr sympathetically with porosity [1] ( Supplementary Fig. S1 ). Similarly, given the temperature dependence of oxygen isotopic fractionation [23] and the temperature increase in burial diagenesis, lower porosity domains are predicted to be depleted in 18 O relative to higher porosity domains, roughly as observed ( Supplementary Fig. S1 ). The emergence of lateral chemical waves seems inevitable as long as a sediment stratum is subjected to a vertical loading. This explains why lateral periodic porosity oscillations are common in dolomite. The proposed mechanism is expected to operate in all stages of sediment burial diagenesis, and its effect on general rock–water interactions still needs to be clarified. For example, during initial dolomitization of a bed, the stress-induced porosity differentiation should occur both in the limestone domain ahead of a reaction front and in the dolomite domain behind the front as dolomitization proceeds. Field and petrographic observations show that stress or crystallization force has an important role in dolomitization [8] , [24] . How the proposed mechanism affects the overall dolomitization process and modifies the original dolomitization signatures is certainly a topic that warrants further research. The proposed mechanism is expected to operate also in other sedimentary rocks, in particular in limestones and sandstones dominated by compaction and pressure solution diagenesis. Lateral porosity and geochemical variations may characterize such rocks, but to our knowledge no previous workers have ever examined sandstones or limestones dominated by burial diagenesis for such features. The proposed mechanism may also apply to other observations in sandstones. For example, it was found that carbonate concretions in the Great Estuarine Group (Middle Jurassic) sandstones post-date the pressure solution of shell against quartz and feldspar but pre-date further compaction [25] . The concretions may thus be spatially distributed in accordance with our model. Careful mapping of calcite cementation in concretions of the Frontier Formation sandstone in central Wyoming does show lateral periodic variations [26] . The length of the concretions is ~4.2 m, and the width is ~5.3 m. Concretion centres are approximately Poisson distributed within the sandstone. Isotopic data indicate that calcite cement is precipitated near a burial depth of 1.5 km (ref. 26 ). The fraction of calcite cement varies horizontally on scale of a few metres to 10 m. The scale of the pattern is consistent with our model prediction. Our model can be extended to sediments comprising multiple mineral phases with different mechanical competency. We believe that the proposed mechanism may be responsible at least partly for concretion formation in shale [25] . Qualitatively, it works as follows: Carbonate minerals, being more mechanically competent, are expected to be the main framework to support the overlying loading. Carbonate crystals in a clay-rich domain would be subjected to a higher effective stress, causing pressure dissolution. The dissolved species would then diffuse to and precipitate in neighbouring carbonate mineral-rich domains. Similar to the dolomite case, this positive feedback would lead to the formation and the lateral separation of concretions in a shale unit. To fully model such processes, a constitutive model able to account for detailed stress partitioning among different mineral phases will be required [27] , [28] . But, nevertheless, the model presented here allows for a rough estimation of the spacing of the concretions. As indicated in equation (14), the typical scale of the pattern depends on D 0 , k , S , β and φ s . The first three parameters are expected to have similar values to those for the dolomite case. However, the last two parameters could be quite different. A shale formation should have a smaller β value (that is, lower mechanical strength) and a smaller porosity value than a dolomite stratum. Let us assume that the parameters β and φ s are 10 and 3 times smaller than those for dolomite, respectively. The spacing of carbonate concretions in shale is then estimated to range from half a decimetre to a few metres, which is roughly consistent with field observations [25] . The foregoing discussion is focused on the emergence of lateral heterogeneity in a single layer of dolomite. Our model would apply, however, to every layer in a vertical sequence and predicts lateral differentiation of porosity within every layer due to stress-mediated mineral-water interactions during burial diagenesis. The magnitude of each layer's response will depend on the attributes of the layer, including bed thickness, initial porosity, mineralogical composition, hydraulic conductivity and rheology, yet any layer that is subjected to stress should respond and differentiate porosity. Field data [1] , [2] , [4] , [5] show that the vertical variation in average properties of each layer in a dolomite sequence (and all sedimentary rocks for that matter) is related to vertical facies changes, but that the range of variations within different facies is often similar in magnitude. The mechanism proposed herein would be one means for creating those similar intrafacies ranges, and would further suggest that lateral intrafacies ranges that were heretofore considered random variations might, in part, relate to structured and predictable self-organizing chemical waves. A question for future study is whether the porosity differentiations in a set of vertically stacked sediment layers would proceed cooperatively through stress coupling and vertical mass transfer during burial diagenesis. Vertical diagenetic differentiation within or between sediment layers is evident in many sedimentary rocks. For example, stylolites are commonly observed in carbonate rocks. These evenly spaced dissolution seams exhibit complex column-to-socket interdigitations, with the lateral extension up to tens of metres and the interseam spacing up to ~1 m (ref. 29 ). They are usually parallel to bedding, if formed owing to a burial stress, or, in some occasions, oblique to bedding, if caused by a tectonic stress. The formation of stylolites has been attributed to the vertical structural differentiation and mass transfer induced by pressure solution [29] . In principle, vertical mass transfer could occur between two neighbouring sediment layers, further differentiating mineralogical composition between the layers and therefore enhancing pre-existing beddings. This process may partly be responsible for the formation of chert–shale couplets in bedded chert. Major and rare-earth element data from Franciscan assemblage and Claremont Formation bedded chert sequences, along with physical observations such as the presence of rare and highly corroded radiolarians in shale interbeds, suggest a dominantly diagenetic origin of chert–shale couplets [30] , contradicting the traditional depositional theories. By incorporating appropriate sediment rheology and vertical mass transfer, our model will be able to simulate any three-dimensional complexity formed in sedimentary rocks during stress-induced burial diagenesis. Finally, an accurate prediction of the scale and geometry of lateral porosity and permeability variations is of great interest for reservoir engineering. Numerical simulations show that fingering, sweep efficiency and breakthrough time in enhanced oil recovery are sensitive to such variations [2] , [31] , [32] . Such effects may also be important for subsurface carbon dioxide sequestration and storage [33] . A linear stability analysis indicates that horizontal permeability variations may enhance supercritical CO 2 dissolution in deep brine aquifers [34] and dramatically change the qualitative behaviour of the buoyancy flow of CO 2 in such environments [35] . Furthermore, lateral porosity variations may create localized stagnant domains that may affect the transport of chemical species in subsurface environments. Small-scale porosity variations have been found to have a significant impact on radionuclide transport in dolomite formations [36] . Our work indicates that a large portion of such variations may originate from self-organized sediment diagenesis and therefore are probably predictable. Curie principle By expanding the term φ in equation (6) into a Taylor's series, we obtain: In an isotropic medium subject to a vertical uniaxial loading, according to the Curie principle [37] , the influence of a surrounding point ( X ′, Y ′) on the point ( X , Y ) should be also isotropic. That is, replacing X − X ′ with X ′− X or Y − Y ′ with Y ′− Y will not change the scalar texture descriptor and therefore the function value of σ , implying that the second, third and sixth terms on the right-hand side of equation (16) must vanish. Let A and B denote the coefficients of the remaining terms: We then obtain equation (7). Derivation of dispersion equation Let ɛ →0 in equation (9–11)): Linearizing the above equations around the steady-state solution with respect to perturbations δφ , δc and δp , we obtain: Assuming that the perturbations have the form: we obtain the following homogeneous algebraic equations: The condition for a nontrivial solution of is: Solving the equation for ζ , we obtain the dispersion equations (12) and (13). Estimation of pattern scale For a no-flow case ( v =0), from equation (12), we have The preferred wave number ω max can be found by taking : We then have: As φ s m ≪ (1− φ s ) ≈ 1 and β is on the order of unity, we obtain: or The term is added to convert the unit of cm 3 solid to the unit of cm 3 solution. For a flow case with a large v , as ω max ,2 =0 ( Fig. 4 ), from equation (12), we have Similarly, the preferred wave number ω max ,1 can be found by taking : Solving for we obtain: We then have: for a large v . Adding the term to convert the unit of cm 3 solid to the unit of cm 3 solution, we obtain: How to cite this article: Wang, Y. & Budd, D.A. Stress-induced chemical waves in sediment burial diagenesis. Nat. Commun. 3:685 doi: 10.1038/ncomms1684 (2012).